Identification of the PGRMC1 protein complex as the putative sigma-2 receptor binding site The sigma-2 receptor, whose gene remains to be cloned, has been validated as a biomarker for tumour cell proliferation. Here we report the use of a novel photoaffinity probe, WC-21 , to identify the sigma-2 receptor-binding site. WC-21 , a sigma-2 ligand containing both a photoactive azide moiety and a fluorescein isothiocyanate group, irreversibly labels sigma-2 receptors in rat liver; the membrane-bound protein was identified as PGRMC1 (progesterone receptor membrane component 1). Immunocytochemistry reveals that both PGRMC1 and SW120 , a fluorescent sigma-2 receptor ligand, colocalize with molecular markers of the endoplasmic reticulum and mitochondria in HeLa cells. Overexpression and knockdown of the PGRMC1 protein results in an increase and a decrease in binding of a sigma-2 selective radioligand, respectively. The identification of the putative sigma-2 receptor-binding site as PGRMC1 should stimulate the development of unique imaging agents and cancer therapeutics that target the sigma-2 receptor/PGRMC1 complex. Sigma-1 and sigma-2 receptors were initially characterized in the mid-1970s using radioligand-binding studies [1] . Radiolabelled benzomorphans such as [ 3 H](+)-pentazocine bind potently and selectively to sigma-1 versus sigma-2 receptors. Characterization of the sigma-2 receptor has relied on radioligand-binding studies using [ 3 H]DTG (1,3 di- o -tolylguanidine) in the presence of (+)-pentazocine or dextrallorphan to block binding to sigma-1 receptors [1] . The sigma-1 receptor was purified, sequenced and cloned from guinea pig brain in 1996, and shows no sequence homology with any mammalian proteins cloned to date [2] . Ligands binding to the sigma-1 receptor modulate the release of neurotransmitters; several of these compounds have shown promise as antipsychotics, antidepressants and drugs blocking the effects of psychostimulants [3] , [4] . Recent studies indicate that the sigma-1 receptor is expressed in postsynaptic sites, regulates ion channels, and may function as a protein chaperone [5] , [6] , [7] , [8] . To date, the sigma-2 receptor has not been purified, sequenced or cloned. Although its structure is not known, the sigma-2 receptor has been validated as a biomarker for tumour cell proliferation both in vitro and in vivo , and as a target for chemotherapy. Several studies have shown that: the sigma-2 receptor density in proliferative breast cancer cells is about tenfold higher than in quiescent breast cancer cells [9] ; sigma-2 receptor expression is upregulated during the transition from quiescence to proliferation and downregulated during the transition from proliferation to quiescence [10] ; sigma-2 receptor density can be used to determine the proliferative status of solid tumours [11] ; sigma-2 receptor ligands can serve as chemotherapeutics for treating solid tumours [12] , [13] , [14] ; and sigma-2 receptor radioligands can be used to image tumours by positron emission tomography or single-photon emission computed tomography [15] , [16] , [17] , [18] , [19] . However, as the sigma-2 receptor gene has not been cloned, the exact role this receptor has in tumour and normal cell proliferation is currently unknown. Our group has developed sigma-2 selective ligands, including [ 3 H] RHM-1 , [ 125 I]RHM-4 and SW120 to directly identify, locate and quantify this protein using a variety of receptor-binding and molecular imaging techniques [13] , [14] , [15] , [18] , [20] , [21] , [22] . Progesterone receptor membrane component 1 (PGRMC1) is overexpressed in a variety of tumours in comparison with the corresponding normal cells, and thus represents an important biomarker for cancer progression and a potential target for anticancer drugs [23] , [24] , [25] . PGRMC1, which exists in phosphorylated and dephosphorylated states during cancer cell proliferation [26] , regulates cell growth and proliferation through interactions between its Cytochrome b5-binding domain and other potential binding partners, which include Insig-1, PAIR-BP1 and P450 proteins [23] , [27] , [28] , [29] , [30] , [31] . Recent studies suggest that PGRMC1 is a biomarker of cell proliferation and an excellent therapeutic target for inhibiting tumorigenesis [24] , [32] , [33] . Interestingly, proteomic studies also showed that PGRMC1 is expressed in high levels in the proliferative cells of human endometrium [34] . The purpose of the current study was to identify the protein or protein complex that contains the sigma-2 receptor ligand-binding site as the first step in determining the role of this receptor in cell proliferation, and defining a new target for the development of novel tumour imaging agents and cancer therapeutics. Here we describe a novel strategy developed for the identification of the sigma-2 receptor. The sigma-2 receptor photoaffinity probe, WC-21 , an analogue of RHM-1 , contains an azide moiety for the photoaffinity tagging of the sigma-2 receptor, and a fluorescein isothiocyanate group (FITC) for protein visualization. WC-21 was utilized to directly label the sigma-2 receptor-binding site in rat hepatic membrane homogenates. Proteomic studies and consequent studies were carried out to determine the molecular identity of the sigma-2 receptor binding site and if it corresponded to any previously identified proteins. PGRMC1 was identified as the putative sigma-2 receptor binding site. The results of our studies provide strong experimental evidence supporting the localization of the putative sigma-2 receptor binding site within the PGRMC1 protein complex. Photoaffinity labelling and protein identification The synthesis of sigma-2 receptor photoaffinity probe WC-21 is described in detail in the supporting online material ( Supplementary Figs S1–S3 ). WC-21 has high binding affinity for sigma-2 receptors ( K i =8.7 nM) and relatively low binding affinity for sigma-1 receptors ( K i >4,000 nM; Fig. 1a ). WC-21 was incubated with rat liver membrane homogenates, and the WC-21 –protein complex photo-crosslinked. The protein supernatant was enriched and separated by gel electrophoresis ( Fig. 1b ). Western blot analysis revealed a dominant protein band at ~24 kDa that was labelled by FITC-conjugated probe WC-21 ( Fig. 1b ). Labelling of this protein band with WC-21 could be blocked by well-characterized sigma-2 receptor ligands ( Supplementary Fig. S4 ). Proteomic studies of the protein in the ~24 kDa band identified two proteins, the 22 kDa putative progesterone-binding protein and the 25 kDa 25-Dx protein, that share the same genetic name, PGRMC1 . 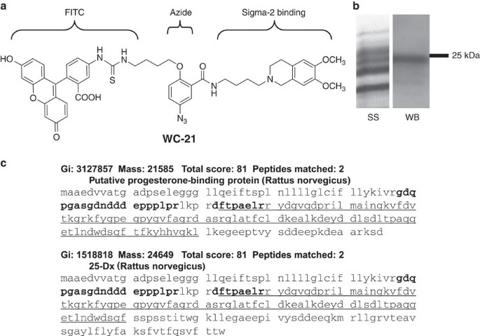Figure 1: Identification of the putative sigma-2 receptor binding site as PGRMC1 using a novel photoaffinity probe. (a)WC-21contains a FITC group and a photoactive azide (N3) moiety, and displays high sigma-2 receptor affinity and selectivity;Ki=8.7±1 nM for sigma-2 receptor andKi>4,000 nM for sigma-1 receptor. (b) Following ultraviolet crosslinking, ligand-labelled proteins were enriched and separated through SDS–polyacrylamide gel electrophoresis;WC-21crosslinked proteins can be visualized using an anti-FITC antibody; SS is silver staining and WB is western blot. (c) Proteomic studies of the FITC-positive band identified two proteins, which shared the same genetic name: progesterone receptor membrane component 1 (PGRMC1). The protein structure shows the peptides (bold) detected by mass spectrometry as well as the Cytochrome b5 domain (underlined). Figure 1c shows the protein sequence of the two peptides, gdqpgasgdndddeppplpr and dftpaelr , detected by mass spectrometry and the Cytochrome b5 domain (underlined) of PGRMC1. The gene for PGRMC1 is located on q22–q24 of the X chromosome [23] . Figure 1: Identification of the putative sigma-2 receptor binding site as PGRMC1 using a novel photoaffinity probe. ( a ) WC-21 contains a FITC group and a photoactive azide (N 3 ) moiety, and displays high sigma-2 receptor affinity and selectivity; K i =8.7±1 nM for sigma-2 receptor and K i >4,000 nM for sigma-1 receptor. ( b ) Following ultraviolet crosslinking, ligand-labelled proteins were enriched and separated through SDS–polyacrylamide gel electrophoresis; WC-21 crosslinked proteins can be visualized using an anti-FITC antibody; SS is silver staining and WB is western blot. ( c ) Proteomic studies of the FITC-positive band identified two proteins, which shared the same genetic name: progesterone receptor membrane component 1 (PGRMC1). The protein structure shows the peptides (bold) detected by mass spectrometry as well as the Cytochrome b5 domain (underlined). Full size image Three other proteins, glutathione- S -transferase alpha type 2, glutathione S -transferase mu 1 (with two matched peptides), and NADH dehydrogenase (ubiquinone) flavoprotein 2 (with one matched peptide), were identified from the proteomics study. Based on the localization of sigma-2 receptors within the plasma membrane [9] , [35] , [36] , endoplasmic reticulum and mitochondria [21] , [22] , these proteins were excluded as potential candidates, as they are all intracellular enzymes, which happen to overlap the PGRMC1 protein band. The pharmacological profile of [ 125 I] RHM-4 in HeLa cells [ 125 I]RHM-4 ( Fig. 2a ) is a useful radioligand for measuring sigma-2 receptor density in tumours and normal tissues [19] . AG-205, a reported PGRMC1 ligand [33] , [37] , and the known sigma-2 receptor ligands, DTG, siramesine, SV119 and WC-26 , readily displaced [ 125 I]RHM-4 binding in HeLa cell membrane homogenates ( Fig. 2a ). Similar results were also observed in mouse mammary 66 tumour cell membrane homogenates ( Supplementary Fig. S5 ). 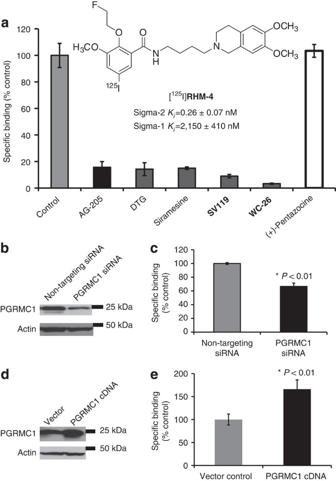Figure 2: The pharmacological profile of [125I]RHM-4 and sigma-2 receptor-binding activity in PGRMC1 siRNA- and cDNA-treated HeLa cells. (a) Competitive binding studies of[125I]RHM-4were carried out with the PGRMC1 ligand AG-205, sigma-2 receptor ligands DTG,WC-26,SV119and siramesine or with the sigma-1 receptor ligand (+)-pentazocine.[125I]RHM-4binding was blocked by AG-205 and the sigma-2 ligands but not by (+)-pentazocine.N=2, sample in triplicate. (b) Typical western blot confirming PGRMC1 protein expression knockdown in PGRMC1-specific siRNA-treated HeLa cells relative to non-targeting siRNA-treated controls compared with actin (loading control). (c) The bar graph shows reduced sigma-2 receptor-binding activity in the PGRMC1 knockdown cells; *P<0.01, Student'st-test,n=3. (d) Typical western blot confirming increased PGRMC1 protein expression in PGRMC1-transfected HeLa cells relative to vector-transfected controls. (e) Bar graph showing increased sigma-2 receptor-binding activity in PGRMC1-transfected cells; *P<0.01, Student'st-test,n=3. Error bars ina,c,erepresent s.e.m. Figure 2: The pharmacological profile of [ 125 I]RHM-4 and sigma-2 receptor-binding activity in PGRMC1 siRNA- and cDNA-treated HeLa cells. ( a ) Competitive binding studies of [ 125 I]RHM-4 were carried out with the PGRMC1 ligand AG-205, sigma-2 receptor ligands DTG, WC-26 , SV119 and siramesine or with the sigma-1 receptor ligand (+)-pentazocine. [ 125 I]RHM-4 binding was blocked by AG-205 and the sigma-2 ligands but not by (+)-pentazocine. N =2, sample in triplicate. ( b ) Typical western blot confirming PGRMC1 protein expression knockdown in PGRMC1-specific siRNA-treated HeLa cells relative to non-targeting siRNA-treated controls compared with actin (loading control). ( c ) The bar graph shows reduced sigma-2 receptor-binding activity in the PGRMC1 knockdown cells; * P <0.01, Student's t -test, n =3. ( d ) Typical western blot confirming increased PGRMC1 protein expression in PGRMC1-transfected HeLa cells relative to vector-transfected controls. ( e ) Bar graph showing increased sigma-2 receptor-binding activity in PGRMC1-transfected cells; * P <0.01, Student's t -test, n =3. Error bars in a , c , e represent s.e.m. Full size image Binding activity in PGRMC1 siRNA and cDNA-treated HeLa cells Because PGRMC1 is a known protein, a number of molecular biology tools are available to study the relationship between the expression of this protein and the binding of sigma-2 selective ligands in cancer cells. Knockdown studies using a PGRMC1-specific short interfering (siRNA; Fig. 2b ) reduced the binding of [ 125 I]RHM-4 to HeLa cells ( Fig. 2c ), indicating that the PGRMC1 complex has binding properties similar to the sigma-2 receptor. Similar results were observed in human embryonic kidney 293T cells using the PGRMC1-specific siRNA and the sigma-2 selective fluorescent probe, SW120 ( Supplementary Fig. S6 ). Cells treated with non-targeting siRNA were used as controls. Overexpression studies were also conducted in HeLa cells using a cDNA for PGRMC1. HeLa cells transfected with the PGRMC1 cDNA displayed an increase in protein levels ( Fig. 2d ) and a 60% increase in binding of [ 125 I]RHM-4 ( Fig. 2e ) over cells transfected with vector alone. Sigma-1 receptor-binding activities, determined using [ 3 H](+)-pentazocine, were found to be not changed in the non-targeting siRNA and PGRMC1 siRNA-treated cells, or in cells transfected with vector and PGRMC1 cDNA ( Supplementary Fig. S7 ). Sigma-2 receptor and PGRMC1 in mammary 66 and 67 cells A good correlation between sigma-2 receptor binding of [ 125 I]RHM-4 and the PGRMC1/actin ratio was observed in mouse mammary adenocarcinoma cells lines 66 and 67 after 6 (proliferative cells), 12 (early quiescent phase) and 18 (late quiescent phase) days in culture ( Supplementary Fig. S8 ). These data are consistent with the expression of sigma-2 receptors in 66 and 67 cells [9] . Caspase-3 activation and PGRMC1 upregulation by WC-26 Studies have shown that sigma-2 receptor ligands can induce caspase-3-dependent cell death [14] , [38] . In the current study, functional assays were conducted to examine the ability of the PGRMC1 to regulate caspase-3 activation by the sigma-2 receptor ligand, WC-26 ( Fig. 3a ). In HeLa cells, knocking down the PGRMC1 resulted in a blunting of the effect of WC-26 to induce caspase-3 activation relative to HeLa cells treated with the non-targeting siRNA ( Fig. 3b ). Also, previous studies have shown that AG-205, a PGRMC1 ligand, induced an upregulation of PGRMC1 in A549 lung cancer cells [33] , [37] . The sigma-2 receptor ligand WC-26 induced an upregulation of PGRMC1 protein in a dose-dependent manner in non-targeting siRNA-treated cells ( Fig. 3c ). Only a minimal increase in PGRMC1 expression was observed in the PGRMC1 knockdown cells. 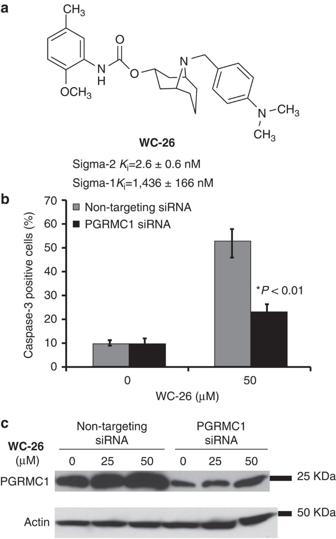Figure 3: Caspase-3 activation and PGRMC1 upregulation induced by the sigma-2 receptor ligand,WC-26. (a) Chemical structure ofWC-26, a selective sigma-2 receptor ligand. (b) Knockdown of PGRMC1 in HeLa cells resulted in decreased caspase-3 activation induced byWC-26. (c)WC-26stimulated PGRMC1 expression in the same manner as AG-205 (ref.34), a PGRMC1 ligand; *P<0.01, Student'st-test,n=3. Error bars inbrepresent s.e.m. Figure 3: Caspase-3 activation and PGRMC1 upregulation induced by the sigma-2 receptor ligand, WC-26 . ( a ) Chemical structure of WC-26 , a selective sigma-2 receptor ligand. ( b ) Knockdown of PGRMC1 in HeLa cells resulted in decreased caspase-3 activation induced by WC-26 . ( c ) WC-26 stimulated PGRMC1 expression in the same manner as AG-205 (ref. 34 ), a PGRMC1 ligand; * P <0.01, Student's t -test, n =3. Error bars in b represent s.e.m. Full size image Intracellular localization of PGRMC1 and sigma-2 receptors The intracellular localization of PGRMC1 and sigma-2 receptors was compared using confocal microscopy. PGRMC1 proteins were visualized with an anti-PGRMC1 antibody, whereas sigma-2 receptors were visualized using the fluorescent probe, SW120 (ref. 21 ; Fig. 4a ). Both the sigma-2 receptor probe ( Fig. 4b,d ) and anti-PGRMC1 antibody ( Fig. 4c,e ) colocalized with markers of the mitochondria ( Fig. 4b,c ) and the endoplasmic reticulum ( Fig. 4d,e ). An additional set of high-magnification images are shown in Supplementary Figure S9 . 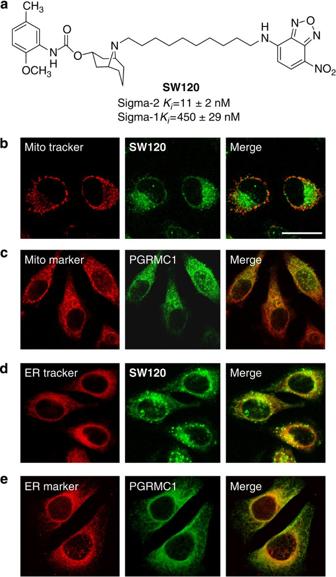Figure 4: Intracellular co-localization of PGRMC1 and sigma-2 receptors in HeLa cells using confocal microscopy. (a) Sigma-2 receptors labelled withSW120and PGRMC1 partially colocalized with mitochondria markers (b,c) and endoplasmic reticulum markers (d,e) in HeLa cells. For imaging sigma-2 receptors, live cells were incubated withSW120and either MitoTracker or ER-Tracker and then imaged by confocal microscopy. For imaging PRGMC1, cells were fixed and incubated with goat anti-PGRMC1 antibody followed by a FITC-conjugated secondary antibody. Antibody stained HeLa cells were then coverslipped and imaged by confocal microscopy. Scale bar represents 20 μm. Figure 4: Intracellular co-localization of PGRMC1 and sigma-2 receptors in HeLa cells using confocal microscopy. ( a ) Sigma-2 receptors labelled with SW120 and PGRMC1 partially colocalized with mitochondria markers ( b , c ) and endoplasmic reticulum markers ( d , e ) in HeLa cells. For imaging sigma-2 receptors, live cells were incubated with SW120 and either MitoTracker or ER-Tracker and then imaged by confocal microscopy. For imaging PRGMC1, cells were fixed and incubated with goat anti-PGRMC1 antibody followed by a FITC-conjugated secondary antibody. Antibody stained HeLa cells were then coverslipped and imaged by confocal microscopy. Scale bar represents 20 μm. Full size image In recent years, considerable effort has been focused on the identification of cancer biomarkers, which could be used in early detection, patient prognosis and prediction of response to different types of chemo- and radiotherapy. In many regards, the sigma-2 receptor possesses a unique ability to serve as both a diagnostic and therapeutic biomarker of solid tumours. The tenfold higher density of sigma-2 receptors in proliferating breast cancer cells versus quiescent breast cells in vitro and in vivo [9] , [11] suggests that measuring the sigma-2 receptor status of solid tumours should provide an assessment of the proliferating/quiescent cell ratio in solid tumours, which could be used by an oncologist to select between certain types of chemotherapy (for example, cell cycle specific versus cell cycle nonspecific) and radiation therapy (hyperfractionated versus conventional radiation therapy). Furthermore, preclinical studies of sigma-2 receptor agonists have shown promise as chemotherapeutic agents, as they are capable of killing tumour cells via a variety of mechanisms including caspase- and non-caspase-mediated apoptosis. However, the widespread acceptance of the sigma-2 receptor as a cancer biomarker has been hampered by the fact that the molecular identity of this protein was not known. The goal of the current study was to complete a series of steps aimed at determining the molecular identity of the sigma-2 receptor. The first step involved the development of a sigma-2 selective photoaffinity probe, which could irreversibly tag sigma-2 receptors in rat liver membrane homogenates, the tissue source used in sigma-2 receptor-binding assays. The photoaffinity labelling and mass spectrometry sequence analysis indicated that a strong candidate protein for the sigma-2 receptor was PGRMC1. A review of the literature revealed a number of similarities between the expression of PGRMC1 in cancer cells and normal tissues, and the density of sigma-2 receptors in the same cancer cells and tissues. The availability of siRNA, cDNA and monoclonal antibodies for PGRMC1 provided the tools needed to study the relationship between the expression of this protein and the binding of sigma-2 selective ligands in cancer cells. The intracellular localization of PGRMC1 and sigma-2 receptors in mitochondria and endoplasmic reticulum, reduction in sigma-2 receptor-binding and caspase-3-mediated cell deaths in PGRMC1 siRNA-treated HeLa cells, and the increase in sigma-2 receptor binding upon overexpressing the PGRMC1 clearly demonstrate that sigma-2 receptor ligands bind to the PGRMC1 protein complex. Therefore, this study is the first to report that the putative sigma-2 receptor ligand-binding site is located within the PGRMC1 protein complex. In addition, the observations that AG-205, a reported PGRMC1 ligand, displaces [ 125 I]RHM-4 from HeLa cell membrane homogenates, and that both AG-205 and the sigma-2 receptor ligand WC-26 induce an upregulation of the PGRMC1 protein in lung cancer cells [33] , [37] and HeLa cells further support our conclusions. The identification that the putative sigma-2 receptor binding site resides within the PGRMC1 protein complex is significant for many reasons. First, it provides a link between receptor-binding studies using sigma-2 radioligands and a known protein, the PGRMC1, which has been validated as a biomarker of cancer and cell proliferation. Second, it provides a gene whose expression can be examined across a wide panel of tumour cells. The genetic mutations and single-nucleotide polymorphism of PGRMC1 can also be readily examined in assessing the possible roles of this gene in normal cell function and in malignant transformation. Finally, the results reported here provide an important scientific bridge between the sigma-2 receptor and the PGRMC1, and make available a variety of radioligands, fluorescent probes and potential small molecule ligands to study the sigma-2 receptor/PGRMC1 complex in solid tumours and cancer cells using a variety of experimental techniques. Chemical synthesis of the compounds and radiotracers The tritiated compound, [ 3 H]RHM-1, was made by American Radiolabelled Chemicals, Inc. via O -alkylation of the corresponding phenol precursor [17] , [20] ; the specific activity of the radioligand was 80 Ci mmol −1 . [ 3 H](+)-Pentazocine was purchased from Perkin-Elmer. [ 125 I]RHM-4 was prepared by an iododestannylation reaction of the corresponding tributyltin precursor [13] , [19] . SV119 , SW120 and WC-26 , and siramesine were synthesized by our group according to published methods [12] , [21] , [39] , [40] . The synthesis of the novel FITC-conjugated probe, WC-21 ( Supplementary Figs S1–S3 ), is described in the Supplementary Methods . AG-205 was purchased from TimTec. DTG and (+)-pentazocine were purchased from Sigma Aldrich. Haloperidol was purchased from Tocris Bioscience. PGRMC1 recombinant protein was purchased from Assay Designs, Inc. Cell membrane and hepatic membrane homogenates Human HeLa and human embryonic kidney 293T cells were grown in minimum essential media (MEM) containing 10% fetal bovine serum, 2 mM L -glutamine, 1% nonessential amino acids and 1× penicillin/streptomycin at 37 °C in a humidified 5% CO 2 /95% air atmosphere. The mouse mammary tumour 66 cells were grown as previously described [9] . The cells were harvested from T75 flasks after 6, 12 or 18 days in culture. For binding assays, cells were mechanically scraped, rinsed with ice-cold phosphate-buffered saline (PBS), transferred to a 15 ml conical centrifuge tube and centrifuged for 10 min at 200 g . The cell pellet from each T75 flask was resuspended in 1 ml of 50 mM Tris-HCl at pH 8.0, and homogenized using an Ultra-Turrax T8 polython homogenizer (IKA Works, Inc.) at speed 3 for 20 s. Hepatic cell membrane homogenates were prepared from the liver of male Sprague–Dawley rats, as previously described [20] . Photoaffinity labelling and protein identification For photoaffinity labelling, 100 nM of WC-21 was incubated in a 96-well plate with rat liver membrane homogenates (~300 μg of protein in a volume of 150 μl) for 1 h, then the reactions were stopped and filtered into 96-well filter plate after being washed three times. The washed filters were irradiated with 254-nm ultraviolet light for 2 min at a distance of 1 cm; the protein-loaded filters were then punched out, pooled and crushed by homogenization in 2% SDS solution in a 15-ml centrifuge tube, following a centrifugation of 10 min at speed of 800 g , the supernatant was mixed with protein gel sample buffer and boiled for 2 min. For western blot analysis of the WC-21 -labelled protein band, lysates containing 35 μg of protein were run on a 12% acrylamide gel and transferred to a polyvinylidene fluoride membrane (Bio-Rad Laboratories). The position of the predominant band of the ligand-labelled protein in the gel was determined using a horseradish peroxidase-conjugated goat anti-FITC antibody (Biodesign International Inc.) at a 1:1,000 dilution ( Supplementary Fig. S3 ). Western blot analysis with a horseradish peroxidase (HRP)-conjugated anti-FITC antibody revealed the predominant protein band at ~24 kDa was labelled by WC-21 ( Fig. 1b ). This protein band labelling could be blocked by sigma-2 receptor ligands, such as DTG, haloperidol and RHM-1 ( Supplementary Fig. 3 ). The 24 kDa band on the silver stained gel was excised and trypsinized; the trypsinized protein solution was further confirmed as tagged with WC-21 an antibody specific for FITC. Proteomic study of the protein solution identified two proteins, the 22-kDa putative progesterone-binding protein and the 25-kDa 25-Dx protein, which share the same genetic name, PGRMC1. For sequencing studies, proteins were enriched by SDS–polyacrylamide gel electrophoresis on 4–15% gradient gels using ~100 μg of protein per loading well. Ten gel pieces containing proteins ranging from 20–26 kDa molecular weight were excised and subjected to electro-elution with Midi GeBAflex-tube (Gerard Biotech). The eluted protein samples were dialyzed with 7,000 MWCO SnakeSkin pleated dialysis tubing (Pierce Biotechnology, Inc.) and lyophilized; the enriched protein sample was further separated with two 12% gels. One gel was silver stained for protein band visualization using a Mass spectrometry compatible kit from Bio-Rad Laboratories and the other gel was transferred to a polyvinylidene fluoride membrane for western blot analysis with a HRP-conjugated anti-FITC antibody ( Fig. 1b ). The FITC-positive protein band was found at molecular weight of 24 kDa, which was determined using the protein standards. The 24 kDa band was excised and trypsinized. Matrix-assisted laser desorption/ionization–mass spectrometry analysis of the trypsinized proteins was performed by the Proteomics and Mass Spectrometry facility of the Donald Danforth Plant Science Center to identify the proteins. PGRMC1 siRNA treatment HeLa cells were plated on 6-well plates at a cell density of 1.5×10 5 cells per well. At 24 h after plating, the cells were treated with either non-targeting siRNA (catalogue number D-001210-02-20, Thermo Scientific Dharmacon, Inc.) or human PGRMC1 siRNAs (catalogue number L-010642-00-0020, Thermo Scientific Dharmacon, Inc.) mixed with DharmaFECT 2 Transfection Reagent (Thermo Scientific Dharmacon, Inc.) to yield a final concentration of 50 nM. siRNA transfection was performed according the siRNA transfection protocol outlined by Dharmacon. At 48 h after siRNA treatment, cells were collected for the sigma-2 receptor-binding assay. The silencing of PGRMC1 was confirmed by western blot analysis. Overexpression of PGRMC1 HeLa cells were plated in 100-mm dishes at 1.5×10 6 per dish. At 24 h after plating, the cells were transfected with the pCMV6-XL4 vector only or human PGRMC1 cDNA (OriGene Technologies, Inc.) using a Fugene 6 transfection reagent (Roche Applied Science). Transfection was carried out according to the guidelines of the manufacturer. For transfection of HeLa cells, 18 μl of Fugene 6 and 10 μg human PGRMC1 cDNA were used. After 24 h, the cells were collected for the sigma-2 receptor-binding assays. The overexpression of PGRMC1 was confirmed by western blot analysis. Caspase-3 activation assay WC-26 -induced caspase-3 activation in PGRMC1 siRNA-treated HeLa cells was quantified by flow cytometry using a FACScan (BD Biosciences) equipped with an air-cooled argon laser. HeLa cells were fixed in 70% ethanol, washed twice with PBS, and incubated with rabbit anti-cleaved-caspase-3 antibody (Cell Signaling Technology) at a 1:50 dilution in BD Perm/Wash buffer (BD Biosciences) for 2 h at 37 °C. The cells were washed three times with PBS, and then incubated with phycoerythrin-conjugated donkey anti-rabbit IgG (BD Biosciences Pharmingen; 1:300 dilution) for 1 h at room temperature. After washing with PBS, 5 μl of 7-amino-actinomycin D (7-AAD, BD Biosciences) was added at a concentration of 0.25 μg of 7-AAD per 1×10 6 cells. The phycoerythrin-conjugated antibody was excited at 488 nm, and the emission collected using a 570 nm filter. The 7-AAD was excited at 488 nm, and the emission collected using a 650-nm long-pass filter. Immunocytochemistry of sigma-2 receptors and PGRMC1 MitoTracker Red CMXRos and ER-Tracker Red dye were purchased from Invitrogen Corporation. HeLa cells were plated in 35-mm diameter glass-bottom dishes at 2×10 5 cells per dish for 24 h. The live cells were incubated with 30 nM SW120 and either the mitochondria tracker, MitoTracker Red CMXRos (20 nM), or the endoplasmic reticulum tracker, ER-Tracker Red (500 nM), for 2 h at 37 °C. The labelled cells were then coverslipped and imaged by confocal microscopy, as previously described [21] , [22] . The images were acquired using a confocal laser scanning microscope (LSM5 Pascal, Carl Zeiss). SW120 was excited using the 488 nm line from an argon laser, and the emission collected through a 505–530 nm band-pass filter. MitoTracker and ER-Tracker were excited using the 543 nm line from a helium–neon laser, and the emission collected through a 560-nm long-pass filter. For imaging PRGMC1, fixed HeLa cells were incubated with goat anti-PGRMC1 antibody at a 1:100 dilutions in the blocking serum overnight at 4 °C. After washing, the cells were incubated with FITC-conjugated donkey anti-goat IgG secondary antibody for 1 h. Rabbit anti-COX IV antibody (Cell signaling) and rabbit anti-GRP78 BiP antibody (Abcam) were used for imaging Mito-marker and ER-marker, respectively. The secondary antibody used for imaging Mito-marker and ER-marker is TRITC-conjugated donkey anti-rabbit IgG. The FITC and TRITC antibody-labelled cells were then coverslipped and imaged by confocal microscopy. Methods for receptor-binding assay, western blot analysis of PGRMC1, real-time PCR for PGRMC1 mRNA expression and synthesis of the novel photoaffinity probe WC-21 and the 1 H nuclear magnetic resonance and 13 C nuclear magnetic resonance spectra for compounds 2 , 3 , 4 , 5 and WC-21 ( Supplementary Figs S10–S19 ) are detailed in the Supplementary Information . How to cite this article: Xu, J. et al . Identification of the PGRMC1 protein complex as the putative sigma-2 receptor-binding site. Nat. Commun. 2:380 doi: 10.1038/ncomms1386 (2011).